Surface-passivated GaAsP single-nanowire solar cells exceeding 10% efficiency grown on silicon Continued development of high-efficiency multi-junction solar cells requires growth of lattice-mismatched materials. Today, the need for lattice matching both restricts the bandgap combinations available for multi-junctions solar cells and prohibits monolithic integration of high-efficiency III-V materials with low-cost silicon solar cells. The use of III-V nanowires is the only known method for circumventing this lattice-matching constraint, and therefore it is necessary to develop growth of nanowires with bandgaps >1.4 eV. Here we present the first gold-free gallium arsenide phosphide nanowires grown on silicon by means of direct epitaxial growth. We demonstrate that their bandgap can be controlled during growth and fabricate core-shell nanowire solar cells. We further demonstrate that surface passivation is of crucial importance to reach high efficiencies, and present a record efficiency of 10.2% for a core-shell single-nanowire solar cell. Improving the cost/efficiency ratio of III-V-based multi-junction cells can be done through efficiency enhancements, by adding additional junctions to the cell stack [1] or through the lowering of cost by replacing the expensive germanium substrate with silicon. Integrating III-V semiconductors and silicon requires overcoming their differences in lattice parameters and thermal expansion coefficient, as well as their polar/non-polar interfaces [2] , [3] . When constrained to a silicon-bottom cell, the optimum dual-junction solar cell, the simplest multi-junction solar cell, has a theoretical 1-sun peak efficiency between 33 and 43% ( [4] , [5] ) when combined with a 1.7 eV bandgap top cell; this can be achieved with a III-V semiconductor consisting of GaAs 0.8 P 0.2. The small contact interface between the nanowire and the silicon substrate ensures that strain from lattice mismatch is relaxed within the first few monolayers [6] . Using the method of gallium (Ga)-assisted growth, gold-free perfect single crystal, gallium arsenide (GaAs) nanowires have been grown directly on silicon [7] . Higher bandgap gallium phosphide (GaP) [8] and gallium arsenide phosphide (GaAsP) [9] , [10] nanowires have also been grown, but only using gold as growth catalyst. Gold is incompatible with silicon [11] , and has been shown to incorporate into the III-V crystal [12] and degrade the optoelectronic properties of the nanowires [13] . In addition, a sparse array of nanowires can absorb almost all incoming light [14] , meaning that only minute amounts of the expensive III-V material is needed for making a nanowire top cell. Devices consisting of a contacted ensemble of free-standing nanowires have been exposed to temperature changes of up to 200 K, demonstrating that their strain-relieving ability is able to overcome the difference in thermal expansion [15] . To fully utilize their advantage with regards to non-lattice-matched growth, the nanowires themselves must also be able to function well as solar cells. Ga-assisted GaAs 0.8 P 0.2 nanowire growth High-quality GaAsP nanowires were grown without the use of a buffer layer on epi-ready Si(111) substrates having a native oxide surface layer. Solid-source molecular beam epitaxy (MBE) was used for the growths. The Ga-assisted vapour–liquid–solid growth method demonstrated with GaAs nanowires [7] , [16] was adapted to allow for the difference in nucleation energy caused by the addition of P to the growth environment. Direct substitution of an As beam flux with a similar P beam equivalent pressure, resulted in a high nucleation rate that caused the Ga droplet to disappear. By lowering the V/III flux ratio, the nucleation rate was decreased and the Ga droplet maintained throughout the nanowire growth ( Fig. 1a ). The growth parameters: V/III flux ratio, P/As flux ratio and temperature, yielding the highest crystal quality, were determined by inspecting the wires using transmission electron microscopy ( Fig. 1b and Supplementary Figs S1–S3 ). The different diffusion lengths and incorporation rates of P and As, in combination with the changing growth landscape, mean that the P/As flux ratio needs to be adjusted throughout the growth ( Fig. 1c ). We were able to grow nanowires with constant P content as well as graded nanowires with P content varied from x =0.15 to x =0.70 (GaAs 1− x P x ) along the wire axis ( Supplementary Fig. S4 ). With a systematic focus on the growth parameters, Ga-assisted GaAs 0.8 P 0.2 nanowires with a 1.7 eV bandgap consisting of a close to perfect zinc-blende crystal were successfully produced. The bandgap of nanowire ensembles was determined using room temperature photoluminescence (PL) and further verified on individual nanowires by energy-dispersive X-ray spectroscopy ( Supplementary Figs S4 and S5 ). 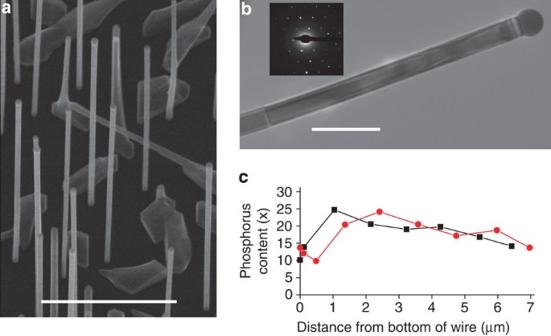Figure 1: Ga-assisted GaAs1−xPxnanowires grown directly on silicon. (a) Scanning electron microscope image of GaAsP nanowires, each having a Ga droplet on top. The nanowires are seen from above at an angle of 25°. Scale bar, 1 μm. (b) Transmission electron microscope image showing the upper part of a GaAsP nanowire with only a few twinnings visible just below the Ga droplet and further down the nanowire. Scale bar, 200 nm. Inset: diffraction image showing the nanowires zinc-blende crystal structure, expanded inSupplementary Fig. S3. (c) Energy-dispersive X-ray spectroscopy characterization of P content (x-value) in two nanowires from the same growth. The variation in P during the first 1 μm of the growth is due to a deliberate flux change, whereas the downward slope is under a constant flux. Figure 1: Ga-assisted GaAs 1− x P x nanowires grown directly on silicon. ( a ) Scanning electron microscope image of GaAsP nanowires, each having a Ga droplet on top. The nanowires are seen from above at an angle of 25°. Scale bar, 1 μm. ( b ) Transmission electron microscope image showing the upper part of a GaAsP nanowire with only a few twinnings visible just below the Ga droplet and further down the nanowire. Scale bar, 200 nm. Inset: diffraction image showing the nanowires zinc-blende crystal structure, expanded in Supplementary Fig. S3 . ( c ) Energy-dispersive X-ray spectroscopy characterization of P content ( x -value) in two nanowires from the same growth. The variation in P during the first 1 μm of the growth is due to a deliberate flux change, whereas the downward slope is under a constant flux. Full size image Core-shell nanowire solar-cell fabrication Solar-cell structures were made by fabricating p–i–n core-shell GaAsP nanowires. The core-shell p–i–n-junction growth method allows for the design of optimal doping densities and layer thicknesses. Further, the radial p–i–n junction ensures a sufficient optical absorption length while minimizing the carrier-extraction distance. First, a p-type core nanowire was grown by introducing beryllium during the axial vapour–liquid–solid growth. A Ga-free step was added to let the group V material consume the Ga droplets and halt further axial growth. Then, two GaAsP shells were grown around the As-grown nanowires, using vapour–solid (VS) epitaxial growth, the first one intrinsic and the second one n-type by doping with silicon. Before the radial shell growth, the substrate temperature was lowered to avoid beryllium diffusion and to enhance n-type doping of the silicon. As and P have different incorporation rates during planer (VS) film growth, and these rates further depend on beam fluxes and growth temperature. To grow a lattice-matched shell around the core nanowire, a series of core-shell growths were carried out to optimize the growth parameters. The growths were characterized using X-ray diffraction, which shows mismatched lattice sizes as multiple peaks in the data plot. For the ideal core-shell nanowire growth, only two peaks should be visible, one from the silicon crystal lattice in the substrate and one from the GaAsP core-shell nanowire. The first growth (R19) in the series had a too high P content in the shell ( Fig. 2a ). The final growth (R22) in the series showed only one III-V peak, indicating a lattice-matched core and shell. The GaAs 0.8 P 0.2 (111) peak should yield a 2Θ≈27.5°, which correlates well with the R22 growth. 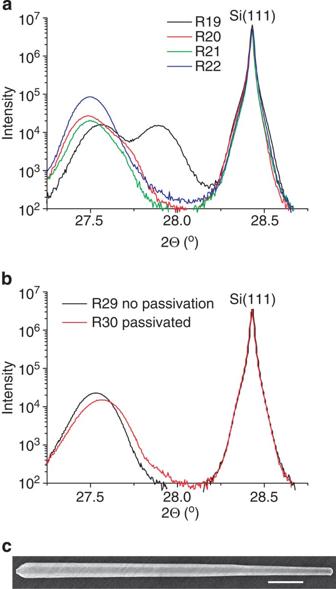Figure 2: Lattice matching of the GaAs1-xPxshell using X-ray diffraction. (a) A GaAsP core-shell growth series consisting of four growths with identical core growth parameters. The series was aligned using the sharp Si(111) peak from the substrate. The peaks to the left are from the nanowire crystal, and any shift or broadening of the peaks towards the right represents a shift in lattice size towards a higher P content. (b) Two GaAsP core-shell growths with the only difference being the addition of an InGaP passivation layer to R30. The unpassivated and passivated SNWSCs were fabricated using nanowires from these two growths. (c) Scanning electron microscope image of a core-shell GaAsP nanowire from the same growth as the best device. Scale bar, 1 μm. Figure 2: Lattice matching of the GaAs 1- x P x shell using X-ray diffraction. ( a ) A GaAsP core-shell growth series consisting of four growths with identical core growth parameters. The series was aligned using the sharp Si(111) peak from the substrate. The peaks to the left are from the nanowire crystal, and any shift or broadening of the peaks towards the right represents a shift in lattice size towards a higher P content. ( b ) Two GaAsP core-shell growths with the only difference being the addition of an InGaP passivation layer to R30. The unpassivated and passivated SNWSCs were fabricated using nanowires from these two growths. ( c ) Scanning electron microscope image of a core-shell GaAsP nanowire from the same growth as the best device. Scale bar, 1 μm. Full size image Single-nanowire solar cell (SNWSC) characterization To produce SNWSCs, the nanowires were removed from the growth substrate, placed on an oxide covered silicon substrate and contacted at both ends (see Fig. 3c and Methods for details on the fabrication scheme). The SNWSCs were characterized individually by measuring current-voltage curves in the dark and under AM1.5G illumination. The best unpassivated SNWSC had an efficiency of 6.8%, short circuit current I SC =13.2 mA cm −2 , open circuit voltage V OC =0.76 V and fill factor (FF)=0.68 ( Fig. 3a ). This efficiency is higher than what has previously been reported [17] , [18] , [19] , but still considerably lower than the theoretical Shockley–Queisser limit, which for a 1.7 eV bandgap is 29%, I SC ~23 mA cm −2 , V OC ~1.4 V and FF~0.9 ( [20] ). For a device geometry similar to ours, it is predicted that roughly half of the projected sunlight is absorbed [21] , which accounts well for the discrepancy between measured and Shockley–Queisser I SC . The measured V OC is also about half of the Shockley–Queisser limit, but this cannot be accounted for by the low absorption in this solar-cell geometry. A low V OC is often attributed to non-optimal doping of the n- and p-region or inadequate surface passivation. 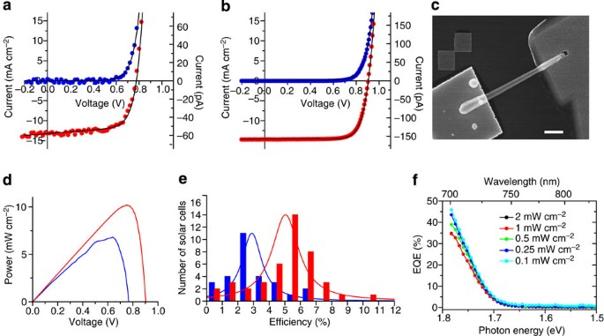Figure 3: Characterization of SNWSCs with and without passivation. (a,b) I-V characteristics under dark (blue dots) and AM1.5G illuminated conditions (red dots) of (a) the unpassivated and (b) passivated SNWSCs with the highest efficiency. The black line is a fit to the data. Passivation increased the efficiency by 50%. (c) A scanning electron microscope image of the best passivated device. Scale bar, 1 μm. (d) P–V comparison between the best passivated (Pmax=10.2 mW cm−2) (red) and unpassivated (Pmax=6.8 mW cm−2) (blue) SNWSC. (e) Histogram of the 1-sun efficiency of 28 unpassivated (blue) and 43 passivated (red) SNWSCs. The Lorentzian fit shows that the passivation has increased the average efficiency by 72% (5.0% for the passivated versus 2.9% for the unpassivated). (f) External quantum efficiency (EQE) versus photon energy of the SNWSC inb,c. Figure 3: Characterization of SNWSCs with and without passivation. ( a , b ) I-V characteristics under dark (blue dots) and AM1.5G illuminated conditions (red dots) of ( a ) the unpassivated and ( b ) passivated SNWSCs with the highest efficiency. The black line is a fit to the data. Passivation increased the efficiency by 50%. ( c ) A scanning electron microscope image of the best passivated device. Scale bar, 1 μm. ( d ) P–V comparison between the best passivated (P max =10.2 mW cm −2 ) (red) and unpassivated (P max =6.8 mW cm −2 ) (blue) SNWSC. ( e ) Histogram of the 1-sun efficiency of 28 unpassivated (blue) and 43 passivated (red) SNWSCs. The Lorentzian fit shows that the passivation has increased the average efficiency by 72% (5.0% for the passivated versus 2.9% for the unpassivated). ( f ) External quantum efficiency (EQE) versus photon energy of the SNWSC in b , c . Full size image Surface passivation Because nanowire solar cells have a high surface to volume ratio compared with planar solar cells, it is critical to passivate the surface of the wires, that is, stopping charge carriers from reaching the surface and recombining at surface states. Simulations on InP core-shell nanowires predicted a 32% improvement in efficiency when reducing the surface recombination [22] . By growing an additional shell of ~10 nm highly n-doped InGaP, we have for the first time applied surface passivation to III-V nanowire solar cells ( Fig. 2b ). The clear faceting in Fig. 2c is a signature of a highly crystalline core-shell growth. Using the passivated nanowires, SNWSCs similar to the unpassivated ones were fabricated. Because the rate of surface recombination typically increases rapidly with bias, introducing a surface-passivation layer should give a large increase in V OC and only a small increase in I SC , which is precisely what we observe ( Fig. 3b ). Another typical sign of a high recombination rate is a low FF and a high ideality factor. The passivation layer increased the fill-factor from 0.68 to 0.77 and decreased the ideality factor from 2.2 to 2.0, indicating that we indeed have lowered the rate of surface recombination ( Table 1 ). With the introduction of a passivation layer, we have been able to significantly increase the peak efficiency to >10% and the average efficiency by 72% ( Fig. 3d ). Characterization as a function of laser wavelength further confirms a 1.7-eV bandgap, because the external quantum efficiency is zero below the bandgap of the nanowire and increases sharply around 1.7 eV ( Fig. 3f ). Table 1 Key performance parameters of the three best passivated and unpassivated SNWSCs Full size table Our realization of GaAsP semiconductor structures directly on silicon, and the excellent performance of the SNWSCs, demonstrates essential steps towards a robust high-efficiency and low-cost dual-junction solar cell. Furthermore, this record SNWSC efficiency has been achieved despite the less than optimal bandgap of GaAsP as a single-junction cell. We still need to optimize the individual nanowires to reach efficiencies close to the Shockley–Queisser limit. We have here demonstrated the first attempt on optimizing the open circuit voltage and FF by means of surface passivation, but have yet to focus on doping concentrations and layer thicknesses in the p–i–n junction. There are additional challenges towards a dual-junction nanowire/planar solar cell. For homogeneous growth and light management, the nanowires should be grown in a positioned array [23] and contacted [24] . The nanowire array must furthermore be produced without any parasitic bulk growth between the nanowires, which will function as Shockley Read Hall recombination centres. The array must be grown on a (111) silicon solar cell, and a tunnel junction must be implemented between the two junctions. The GaAsP/Si dual-junction solar cell is only one example of how nanowires can be used to produce more cost-efficient multi-junction solar cells in the future. The inherent ability of nanowires to relieve strain while conserving crystal quality means that lattice matching between two or more of the solar-cell junctions can be relaxed, thereby allowing for new and better bandgap combinations to be used. Our growth method should enable growth of nanowires in the full 1.42–2.26 eV GaAsP bandgap range, which could facilitate their use as both the top junction in a III-V on Si dual-junction solar cell and a fourth junction in a four-junction solar cell. In conclusion, we have demonstrated high-quality gold-free GaAsP nanowires, grown directly on silicon, with an optimum bandgap for use in a dual-junction silicon-based solar cell. The nanowires have intrinsic properties that overcome the requirements for lattice matching, as well as the difference in thermal expansion coefficient and polar/non-polar interface, which until now have hampered III-V on silicon growth. A surface-passivated GaAsP SNWSC has achieved a 1-sun record efficiency of 10.2%, which effectively doubles the previous SNWSC record [17] , [18] , [19] . Crystal growth The GaAsP core-shell nanowires were fabricated using solid-source III-V MBE. Substrates of 380-μm thick B-doped Si(111) with a thin layer of native oxide were used in the experiments. To enhance the reproducibility between growths, the substrates were first heated to 1100 °C in the MBE system to remove the existing layer of surface oxide, and afterwards kept for 24 h in the clean room before being re-loaded into the MBE system. Using the method of Ga-assisted growth, the core nanowires were grown by means of a Ga droplet that formed on the silicon surface during the first few seconds of the growth procedure. The core-nanowire growths were carried out at a substrate temperature ranging between 620 and 650 °C measured using a pyrometer. For the core growth series, the Ga flux was varied between the growths but kept within the range of 4 × 10 −8 –9 × 10 −8 torr. The group V flux was also varied between growths but was within the range of 2.8 × 10 −6 –7.0 × 10 −6 torr. Core-nanowire growth times were up to 1 h. Following core-nanowire growth, the Ga shutter was closed to interrupt axial growth. During the 10–20 min growth interrupt, the Ga droplets were consumed by the group V fluxes, and the temperature was lowered to 460–470 °C where shell growth was carried out. For p-type doping of the core, a Be doping density corresponding to 8 × 10 17 cm −3 for planar growth of GaAs at 1 ML s −1 was used, and for the n-type shell growth, a silicon doping density corresponding to 0.8 × 10 18 –1.3 × 10 18 cm −3 for planar growth at 1 ML s −1 was used. Device fabrication The wires were removed from the growth substrate by sonication in isopropanol and drip dried onto strongly p-doped Si(100) substrates covered with 500 nm thermal SiO 2 and pre-fabricated alignment marks. The contact to the p-doped core was defining using e-beam lithography followed by a 45–60 s etch at 30 °C in H 3 PO 4 :H 2 O 2 :H 2 O (1:1:15) to expose the core and subsequent thermal evaporation of 5 nm Au/30 nm Zn/150 nm Au. The p-contact was annealed for 2 min at 420 °C in a N 2 atmosphere. Contact to the n-doped wire surface was defined using e-beam lithography followed by a 20 s B-HF etch to remove oxide and a quick load into the evaporation chamber. Several n-contacts have been tested. The results in this article have been achieved with unannealed 40 nm Ge/60 nm Au/27 nm Ni/200 nm Au, annealed 100 nm Ge/100 nm Au for 2 min at 300 °C in a N 2 atmosphere and annealed 6 nm In/240 nm Au-Ge eutectic for 2 min at 300 °C in a N 2 atmosphere. Contact pads were defined using ultraviolet lithography and consist of e-beam evaporated 10 nm Ti/150 nm Au. Optical characterization Solar illumination was done with a standard solar simulator (LOT—Oriel 150 W Xe lamp) with a 1′ beam diameter and an AM1.5G filter. The 1-sun intensity was verified using a mono-crystalline silicon solar cell calibrated at Radboud University Nijmegen against a National Renewable Energy Laboratory (NREL) secondary cell standard. For the quantum efficiency measurements, a continuous wave titanium sapphire laser, tuneable from 700 to 1000, nm, was used. How to cite this article: Holm, J.V. et al . Surface-passivated GaAsP single-nanowire solar cells exceeding 10% efficiency grown on silicon. Nat. Commun. 4:1498 doi: 10.1038/ncomms2510 (2013).